Prostaglandin E2promotes Th1 differentiation via synergistic amplification of IL-12 signalling by cAMP and PI3-kinase T helper 1 (Th1) cells have critical roles in various autoimmune and proinflammatory diseases. cAMP has long been believed to act as a suppressor of IFN-γ production and Th1 cell-mediated immune inflammation. Here we show that cAMP actively promotes Th1 differentiation by inducing gene expression of cytokine receptors involved in this process. PGE 2 signalling through EP2/EP4 receptors mobilizes the cAMP-PKA pathway, which induces CREB- and its co-activator CRTC2-mediated transcription of IL-12Rβ2 and IFN-γR1. Meanwhile, cAMP-mediated suppression of T-cell receptor signalling is overcome by simultaneous activation of PI3-kinase through EP2/EP4 and/or CD28. Loss of EP4 in T cells restricts expression of IL-12Rβ2 and IFN-γR1, and attenuates Th1 cell-mediated inflammation in vivo . These findings clarify the molecular mechanisms and pathological contexts of cAMP-mediated Th1 differentiation and have clinical and therapeutic implications for deployment of cAMP modulators as immunoregulatory drugs. Thelper (Th) 1 cells have critical roles in various inflammatory immune diseases. Differentiation of naive T cells to Th1 cells is driven by two critical cytokines, interleukin (IL)-12 and interferon (IFN)-γ, the former derived from antigen-presenting cells and the latter mainly from T cells, at the beginning, on T-cell receptor (TCR) stimulation [1] . Another cytokine produced on TCR activation, IL-2, is also important in the early stage of Th1 differentiation [2] . TCR ligation initiates activation of Lck and recruitment of ZAP-70 to the TCR complex to generate multiple downstream signals, resulting in the production of cytokines including IL-2 and IFN-γ, upregulation of cell surface molecules such as CD25, and induction of transcription factors for differentiation of Th cells such as T-bet [3] . Prostaglandin E 2 (PGE 2 )-cyclic adenosine monophosphate (cAMP) signalling has long been believed to act as a potent negative regulator of T cells, especially Th1 cells, and is thought to mediate inhibition of immune inflammation in vivo [4] , [5] , [6] , [7] , [8] . It was reported that cAMP inhibits almost all pathways downstream of TCR stimulation and suppresses T cell activation, proliferation and cytokine production [8] . In contrast to this long-believed prevailing view, we and others previously reported that PGE 2 facilitates IL-12-driven Th1 differentiation through its receptor EP2 and EP4 (refs 9 , 10 ), the major downstream signalling of which is a rise in cAMP [11] , and that this PGE 2 action operates in vivo in various mouse models of immune inflammation, such as experimental allergic encephalomyelitis, contact hypersensitivity (CHS), and collagen-induced arthritis. Consistently, genome-wide association studies have revealed that the PTGER4 (encoding human EP4) gene is associated with multiple sclerosis and Crohn’s disease (CD) [12] , [13] , [14] , where the association with IL12RB2 (human IL-12Rβ2), a marker of Th1 cells, was also found [14] , [15] . Furthermore, a recent study shows that T cells deficient in Gαs and, therefore, incapable of producing cAMP, display impaired Th1 differentiation and fail to induce an inflammatory response [16] . While these studies suggest that PGE 2 -cAMP signaling promotes rather than suppresses development of Th1 cells, there are several issues remain to be answered. For example, (1) how is this cAMP action reconciled with its inhibitory effects demonstrated by many previous studies, (2) what is the molecular mechanism whereby cAMP promotes Th1 development and, (3) what is the pathophysiological context in which this cAMP action is used? cAMP activates protein kinase A (PKA) and induces phosphorylation of the transcription factor cAMP responsive element (CRE)-binding protein (CREB) at Ser133. Phosphorylated CREB binds to CRE-containing promoter and initiates gene transcription, usually with its coactivator CREB-binding protein/p300 (ref. 17 ). CREB-dependent gene expression is also promoted by another family of coactivators named cAMP-regulated transcriptional coactivator (CRTC) that binds to CREB in phospho-Ser133-dependent and -independent manners [18] , [19] . Among the three members of the CRTC family, CRTC2 is present in abundance in the liver [18] , spleen and lymph nodes ( http://biogps.gnf.org/ ). Under the basal conditions, CRTC2 is phosphorylated at Ser171 by salt-inducible kinase (SIK) [20] , and sequestered in the cytoplasm. PKA phosphorylates SIK in the C-terminal regulatory domain and inhibits its CRTC kinase activity, which triggers CRTC dephosphorylation and nuclear translocation [21] . While the SIK-CRTC pathway has been shown to be crucial for such physiological processes as gluconeogenesis, neuronal survival and melanogenesis [18] , [19] , [22] , its function in T-cell-mediated immune response has never been reported. IL-12 and IFN-γ act on their cognate receptors to drive differentiation of Th1 cells from naive T cells [1] . The IL-12 receptor is composed of two subunits, β1 and β2 chains (IL-12Rβ1 and β2), among which the latter is induced specifically during Th1 differentiation [23] , [24] and is responsible for IL-12 signal transduction [25] . However, its expression mechanism is not known in detail. Moreover, although naive T cells express both subunits of IFN-γ receptor, α and β chains (IFN-γR1 and R2), IFN-γR1 is downregulated shortly after TCR engagement in vitro [26] . Whether there is any signal counteracting this downregulation of IFN-γR1 by TCR or directly inducing IFN-γR1 expression is currently unknown. Such a signal, if present, may be important, because the downregulation of IFN-γR1 may restrict IFN-γ signalling, which is essential for induction of Th1-lineage-specific transcription factor T-bet and IL-12Rβ2 in the early stage of Th1 differentiation [27] . Here we demonstrate that cAMP promotes Th1 differentiation through upregulation of IL-12Rβ2 and IFN-γR1 and the amplification of these cytokine signalling pathways. PGE 2 mobilizes cAMP-PKA cascade, which directly induces gene expression of IL-12Rβ2 and IFN-γR1 through CREB and CRTC2. Simultaneous activation of PI3K by PGE 2 rescues T cells from the inhibitory effects of cAMP on TCR signalling, and promotes Th1-facilitative action of cAMP by maintaining, for example, production of IL-2 and IFN-γ and expression of CD25. We further report that selective disruption of EP4 signalling in T cells limits expression of the above Th1 cytokine receptors and attenuates Th1-mediated inflammation in vivo . Induction of IL-12Rβ2 in TCR-activated T cells by PGE 2 To clarify how PGE 2 facilitates Th1 differentiation, we examined effects of PGE 2 on expression of IFN-γ ( Ifng ), T-bet ( Tbx21 ), and IL-12Rβ2 ( Il12rb2 ), three genes critical for Th1 differentiation, in T cells cultured under the Th1-priming conditions. PGE 2 considerably enhanced expression of Il12rb2 and Ifng mRNA from 12 and 48 h, respectively, while enhancement of Tbx21 expression was not seen until 72 h ( Fig. 1a ). Enhanced expression of Il12rb2 mRNA at 24 h was mimicked by agonists selective to EP2 (ONO-AE1-259) or EP4 (ONO-AE1-329) but not by agonists to EP1 (ONO-DI-004) or EP3 (ONO-AE-248) (ref. 28 ) ( Fig. 1b ). Induction of IL-12Rβ2 protein by PGE 2 , EP2 or EP4 agonist during Th1 differentiation was confirmed by flow cytometry ( Fig. 1c ). These data suggested that promotion of Th1 differentiation by PGE 2 is likely to be initiated through induction of IL-12Rβ2 via EP2 and EP4 receptors. 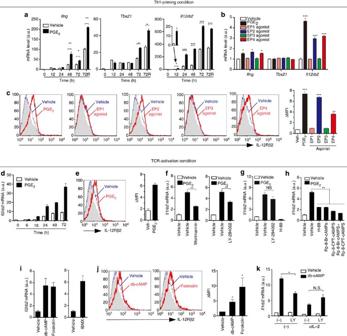Figure 1: PGE2-cAMP signalling induces IL-12Rβ2 expression in TCR-activated T cells. (a) Expression ofIfng,Tbx21andIl12rb2mRNA by T cells activated for indicated times with antibody to CD3 and antibody to CD28 (αCD3/CD28) in the absence or presence of PGE2under Th1-priming conditions. A portion of cells were restimulated with PMA and ionomycin for the last 4 h (72R). (b) Expression ofIfng,Tbx21andIl12rb2mRNA by T cells activated for 24 h with αCD3/CD28 in the absence or presence of PGE2or selective agonists to EP1 to EP4 under Th1-priming conditions. (c) Surface expression of IL-12Rβ2 in T cells activated for 48 h with αCD3/CD28 in the absence or presence of PGE2or agonists selective to EP1 to EP4 under Th1-priming conditions. Grey-filled histogram represents isotype control. ΔMFI (mean fluorescence intensity) indicates the differences between MFI of IL-12Rβ2 and MFI of isotype control (right). (d) Time-course ofIl12rb2mRNA expression by PGE2in T cells activated with αCD3/CD28. (e) PGE2induces IL-12Rβ2 protein expression in T cells activated with αCD3/CD28 for 48 h. (f,g) Expression ofIl12rb2mRNA in WT T cells (f) or IFN-γR1–/–T cells supplemented with anti-IL-2 (g), activated for 24 h with αCD3/CD28 in the absence or presence of PGE2with or without Wortmannin, LY-294002 or H-89. (h) Expression ofIl12rb2mRNA in T cells activated for 24 h with αCD3/CD28 in the absence or presence of PGE2with H-89, Rp-8-Br-CAMPS or Rp-8-CPT-CAMPS. (i,j) Expression of IL-12Rβ2 mRNA (i) and protein (j) in T cells activated with αCD3/CD28 in the presence of db-cAMP, forskolin or 3-isobutyl-1- methylxanthine (IBMX) for 12 h (i) or 48 h (j). (k) Expression ofIl12rb2mRNA in IFN-γR1−/−CD4+T cells activated for 24 h with αCD3/CD28 with or without db-cAMP in the absence or presence of anti-IL-2 or LY-294002 (LY) or both. Data shown as mean±s.e.m. are representative of two or more independent experiments with triplicates. Statistical significance was examined by unpaired two-tailed Student’st-test, *P<0.05; **P<0.01; ***P<0.001. NS, not significant, veh, vehicle; a.u., arbitrary units. Figure 1: PGE 2 -cAMP signalling induces IL-12Rβ2 expression in TCR-activated T cells. ( a ) Expression of Ifng , Tbx21 and Il12rb2 mRNA by T cells activated for indicated times with antibody to CD3 and antibody to CD28 (αCD3/CD28) in the absence or presence of PGE 2 under Th1-priming conditions. A portion of cells were restimulated with PMA and ionomycin for the last 4 h (72R). ( b ) Expression of Ifng , Tbx21 and Il12rb2 mRNA by T cells activated for 24 h with αCD3/CD28 in the absence or presence of PGE 2 or selective agonists to EP1 to EP4 under Th1-priming conditions. ( c ) Surface expression of IL-12Rβ2 in T cells activated for 48 h with αCD3/CD28 in the absence or presence of PGE 2 or agonists selective to EP1 to EP4 under Th1-priming conditions. Grey-filled histogram represents isotype control. ΔMFI (mean fluorescence intensity) indicates the differences between MFI of IL-12Rβ2 and MFI of isotype control (right). ( d ) Time-course of Il12rb2 mRNA expression by PGE 2 in T cells activated with αCD3/CD28. ( e ) PGE 2 induces IL-12Rβ2 protein expression in T cells activated with αCD3/CD28 for 48 h. ( f , g ) Expression of Il12rb2 mRNA in WT T cells ( f ) or IFN-γR1 –/– T cells supplemented with anti-IL-2 ( g ), activated for 24 h with αCD3/CD28 in the absence or presence of PGE 2 with or without Wortmannin, LY-294002 or H-89. ( h ) Expression of Il12rb2 mRNA in T cells activated for 24 h with αCD3/CD28 in the absence or presence of PGE 2 with H-89, Rp-8-Br-CAMPS or Rp-8-CPT-CAMPS. ( i , j ) Expression of IL-12Rβ2 mRNA ( i ) and protein ( j ) in T cells activated with αCD3/CD28 in the presence of db-cAMP, forskolin or 3-isobutyl-1- methylxanthine (IBMX) for 12 h ( i ) or 48 h ( j ). ( k ) Expression of Il12rb2 mRNA in IFN-γR1 −/− CD4 + T cells activated for 24 h with αCD3/CD28 with or without db-cAMP in the absence or presence of anti-IL-2 or LY-294002 (LY) or both. Data shown as mean±s.e.m. are representative of two or more independent experiments with triplicates. Statistical significance was examined by unpaired two-tailed Student’s t -test, * P <0.05; ** P <0.01; *** P <0.001. NS, not significant, veh, vehicle; a.u., arbitrary units. Full size image At least three cytokine signalling pathways, IL-12, IFN-γ and IL-2, are involved in Th1-priming in the culture system we used. Given that all of these cytokines have the ability to induce IL-12Rβ2 in T cells [2] , [24] , [29] , we asked whether these cytokines signalling are involved in PGE 2 -induced IL-12Rβ2 expression. We stimulated T cells with anti-CD3 and anti-CD28 without exogenous IL-12 and found that PGE 2 still upregulated Il12rb2 mRNA and protein expression ( Fig. 1d ). Furthermore, blockade of IL-12 signalling by anti-IL-12 had little effect on the basal or PGE 2 -induced IL-12Rβ2 expression in TCR-activated T cells ( Supplementary Fig. S1a ). Blockade of IFN-γ ( Supplementary Fig. S1b ) or both IFN-γ and IL-2 ( Supplementary Fig. S1c ) signalling by using IFN-γR1 −/− T cells [30] and anti-IL-2 reduced both the basal IL-12Rβ2 expression and its enhancement by PGE 2 . However, even without IFN-γ and IL-2 action, PGE 2 still exhibited enhancement of IL-12Rβ2 expression over the basal level ( Supplementary Fig. S1c ). EP2 and EP4 agonists again mimicked this action of PGE 2 on expression of IL-12Rβ2 mRNA and protein in TCR-activated T cells ( Supplementary Fig. S1d,e ), and the induction of Il12rb2 mRNA expression by EP2 or EP4 agonists was defective in EP2- or EP4-deficient T cells, respectively ( Supplementary Fig. S1f ), confirming that EP2 and EP4 mediate IL-12Rβ2 induction by PGE 2 . Involvement of PI3K and cAMP in PGE 2 -induced IL-12Rβ2 Given that EP2 and EP4 stimulation activates both PI3-kinase (PI3K)-Akt and cAMP-PKA pathways [9] , we examined their involvement in IL-12Rβ2 induction by PGE 2 . Inhibitors of PI3K (LY-294002 and wortmannin) partially prevented PGE 2 -induced Il12rb2 expression in TCR-activated T cells ( Fig. 1f ). As PI3K-Akt pathway mediates TCR-induced production of IFN-γ and IL-2 that have important roles in IL-12Rβ2 expression and Th1 differentiation [2] , [31] , we examined effects of LY-294002 on IL-12Rβ2 induction in TCR-activated IFN-γR1-deficient T cells supplemented with anti-IL-2. Under this condition where both IFN-γ and IL-2 signalling were blocked, LY-294002 did not inhibit PGE 2 -induced Il12rb2 expression ( Fig. 1g ). These results indicate that there are PI3K-dependent and -independent mechanisms of Il12rb2 induction and the former was dependent on IFN-γ and IL-2. Intriguingly, PKA inhibitors (H-89, Rp-8-Br-cAMPS or Rp-8-CPT-cAMPS) [32] also attenuated PGE 2 -induced Il12rb2 expression in TCR-activated wild-type (WT) T cells ( Fig. 1h ), and H-89 completely suppressed IL-12Rβ2 induction in the absence of IFN-γ and IL-2 signalling ( Fig. 1g ). Conversely, expression of IL-12Rβ2 mRNA and protein was enhanced by dibutyryl cAMP (db-cAMP) and forskolin ( Fig. 1i ). Moreover, Il12rb2 mRNA was upregulated by a nonspecific phosphodiesterase (PDE) inhibitor 3-isobutyl-1- methylxanthine ( Fig. 1i ), suggesting that endogenous cAMP has a role in IL-12Rβ2 expression. Interestingly, cAMP-induced IL-12Rβ2 expression in TCR-activated T cells was suppressed partially by PI3K inhibitors but this suppression was not seen when both IFN-γ and IL-2 signalling were blocked ( Fig. 1k ). Direct and indirect induction of IL-12Rβ2 by cAMP As the above results suggest the involvement of IFN-γ and IL-2 in a part of cAMP-induced Il12rb2 expression by TCR-activated T cells, we next evaluated how and how much IFN-γ and IL-2 contribute to cAMP-induced Il12rb2 expression by stimulating T cells with or without TCR activation, with or without IFN-γ signalling, and in the presence or absence of cAMP for 12 h. In WT T cells, while db-cAMP, IFN-γ or TCR activation alone induced Il12rb2 expression at a similar level, cAMP synergistically induced Il12rb2 expression in the presence of IFN-γ or TCR or both ( Fig. 2a ). Addition of anti-IFN-γ did not affect the stimulation by db-cAMP in unactivated T cells, but blunted cAMP response in TCR-activated cells. Consistently, none of the above synergistic effects of IFN-γ or TCR with cAMP was seen in IFN-γR1 −/− T cells at 12 h ( Fig. 2a ). Synergistic action of cAMP with IFN-γ or TCR activation on IL-12Rβ2 protein expression in T cells was also confirmed ( Fig. 2b ). We then evaluated the involvement of IL-2 signalling in cAMP-induced IL-12Rβ2 expression. We used IFN-γR1 −/− T cells to exclude the effect of IFN-γ signalling. Although cAMP and TCR signalling had no synergistic action on Il12rb2 expression in IFN-γR1 −/− T cells at 12 h ( Fig. 2a ), we noted that they synergistically induced Il12rb2 expression after 24 h and this synergistic action was eliminated by anti-IL-2 ( Fig. 2c ), suggesting that synergistic action on Il12rb2 expression with TCR activation and cAMP was mediated by IL-2 and this phenomenon did not appear until 24 h of stimulation. Consistently, blocking either IFN-γ or IL-2 signalling downregulated the basal, as well as the cAMP-induced Il12rb2 expression, and blocking both further reduced Il12rb2 expression in TCR-activated WT T cells at 36 h, but cAMP still enhanced Il12rb2 expression over the basal level under these conditions ( Fig. 2d ). These results demonstrate that there are direct and indirect mechanisms of cAMP-promoted Il12rb2 expression, and that IFN-γ and IL-2 are involved in the latter indirect mechanism. 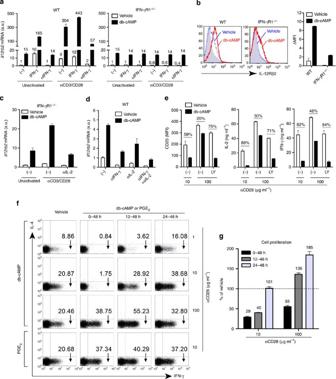Figure 2: cAMP context-dependently regulates TCR activation and Th1 differentiation. (a) Expression ofIl12rb2mRNA in WT (left) and IFN-γR1−/−(right) T cells activated for 12 h without (unactivated) or with αCD3/CD28 in the presence or absence of db-cAMP, IFN-γ or anti-IFN-γ. (b) Surface expression of IL-12Rβ2 in WT or IFN-γR1−/−T cells activated for 48 h with αCD3/CD28. db-cAMP or vehicle was added from 24–48 h. (c) Expression ofIl12rb2mRNA in IFN-γR1–/–T cells activated for 24 h without (unactivated) or with αCD3/CD28 in the absence or presence of db-cAMP or anti-IL-2 or both. (d) Expression ofIl12rb2mRNA in T cells activated with αCD3/CD28 for 36 h with addition of db-cAMP, anti-IFN-γ or anti-IL-2 for the last 12 h. (e) Expression of CD25 and production of IL-2 and IFN-γ by T cells activated with αCD3 and indicated concentrations of αCD28 and treated with db-cAMP or LY-294002 (LY) for 24 h. The percentages indicate the cAMP-mediated inhibition compared with each vehicle group. (f,g) T cells were activated for 48 h with αCD3 and indicated concentrations of αCD28 and treated with db-cAMP or PGE2for indicated periods under Th1-priming conditions. Cells were then washed and reincubated for another 24 h under Th1-priming conditions followed by intracellular staining of IFN-γ (f). Effect of cell proliferation by cAMP is presented as a percentage relative to vehicle group (100%) under each αCD28 condition (g). Data shown as mean±s.e.m. are representative of two independent experiments with triplicates. MFI, mean fluorescence intensity; a.u., arbitrary units. Figure 2: cAMP context-dependently regulates TCR activation and Th1 differentiation. ( a ) Expression of Il12rb2 mRNA in WT (left) and IFN-γR1 −/− (right) T cells activated for 12 h without (unactivated) or with αCD3/CD28 in the presence or absence of db-cAMP, IFN-γ or anti-IFN-γ. ( b ) Surface expression of IL-12Rβ2 in WT or IFN-γR1 −/− T cells activated for 48 h with αCD3/CD28. db-cAMP or vehicle was added from 24–48 h. ( c ) Expression of Il12rb2 mRNA in IFN-γR1 –/– T cells activated for 24 h without (unactivated) or with αCD3/CD28 in the absence or presence of db-cAMP or anti-IL-2 or both. ( d ) Expression of Il12rb2 mRNA in T cells activated with αCD3/CD28 for 36 h with addition of db-cAMP, anti-IFN-γ or anti-IL-2 for the last 12 h. ( e ) Expression of CD25 and production of IL-2 and IFN-γ by T cells activated with αCD3 and indicated concentrations of αCD28 and treated with db-cAMP or LY-294002 (LY) for 24 h. The percentages indicate the cAMP-mediated inhibition compared with each vehicle group. ( f , g ) T cells were activated for 48 h with αCD3 and indicated concentrations of αCD28 and treated with db-cAMP or PGE 2 for indicated periods under Th1-priming conditions. Cells were then washed and reincubated for another 24 h under Th1-priming conditions followed by intracellular staining of IFN-γ ( f ). Effect of cell proliferation by cAMP is presented as a percentage relative to vehicle group (100%) under each αCD28 condition ( g ). Data shown as mean±s.e.m. are representative of two independent experiments with triplicates. MFI, mean fluorescence intensity; a.u., arbitrary units. Full size image cAMP context-dependently regulates Th1 differentiation The above results that cAMP synergizes with IFN-γ and IL-2 in Il12rb2 induction in TCR-activated T cells led us to wonder how such synergistic effects are elicited by cAMP, because cAMP is known to suppress production of these cytokines by inhibiting TCR signalling. We confirmed that cAMP treatment at the beginning of TCR stimulation indeed strongly suppressed markers of T-cell activation such as CD25, IL-2 and IFN-γ. However, this inhibitory effect of cAMP could be rescued by enhancing CD28 costimulation and, intriguingly, this rescue was repressed by LY-294002 ( Fig. 2e ). These results suggest that coactivation of PI3K overcomes the suppression of TCR signalling by cAMP, and allows cAMP to facilitate Il12rb2 expression. We then asked whether similar coactivation of PI3K could rescue cAMP inhibition of Th1 differentiation. To this end, we stimulated T cells with anti-CD3 and different concentrations of anti-CD28 and treated cells with db-cAMP for various periods under Th1-priming conditions. cAMP-mediated inhibition of Th1 differentiation was rescued or overcome by the strengthening CD28 costimulation or by the addition of cAMP at later times after TCR activation, which avoided cAMP-mediated inhibition on initiation of TCR signalling ( Fig. 2f ). Moreover, PGE 2 did not inhibit but promoted Th1 differentiation even if it was added into cultures at the beginning of TCR ligation (0 h) at a CD28 costimulation level where cAMP showed an extremely strong inhibitory effect ( Fig. 2f ). This could be due to the fact that PGE 2 activated both cAMP and PI3K pathways through EP2 and EP4 in T cells [9] and PI3K antagonized cAMP-dependent inhibition of TCR signalling [33] . Similarly, cAMP-mediated inhibition of cell proliferation during Th1 differentiation was also rescued by strengthening CD28 costimulation or postponing cAMP treatment ( Fig. 2g ). Upregulation of IFN-γR1 and IL-2Rβ by cAMP As the above findings suggest that cAMP can induce IL-12Rβ2 expression in T cells partly through IFN-γ and IL-2, the next question was how cAMP amplified IFN-γ and IL-2 signalling. We first noted that the induction of Il12rb2 by cAMP was partially reduced by treatment of the cells with cycloheximide, suggesting the involvement of new protein synthesis in this process ( Fig. 3a ). To identify protein(s) newly synthesized in response to cAMP, we profiled gene expression in TCR-activated WT and IFN-γR1 −/− T cells stimulated with or without db-cAMP. Consistent with previous reports [8] , cAMP inhibited gene expression of several cytokines such as Il2 , Ifng , Tnf and Lta in TCR-activated T cells ( Fig. 3b ). In congruence with our results ( Fig. 2a ), Il12rb2 expression was upregulated by db-cAMP in both WT and IFN-γR1 −/− T cells ( Fig. 3b ), verifying an IFN-γ signalling-independent induction of Il12rb2 by cAMP. Additionally, we noted enhanced expression of genes encoding receptors for IFN-γ and IL-2, such as Ifngr1 and Il2rb , in T cells ( Fig. 3b ). We confirmed by real-time PCR and flow cytometry that cAMP increased both Ifngr1 mRNA and IFN-γR1 protein expression in naive T cells ( Fig. 3c ). This action of cAMP was also observed in TCR-activated T cells, although TCR itself strongly downregulated IFN-γR1 expression ( Fig. 3c ). IFN-γ-induced STAT1 activation in naive T cells was also enhanced by pretreatment with db-cAMP, suggesting that cAMP amplifies IFN-γ signalling ( Fig. 3e ). Similarly, cAMP also upregulated Il2rb mRNA expression in T cells after 24 h, but not 12 h, stimulation ( Fig. 3f ) and upregulation of IL-2Rβ protein expression by cAMP was also confirmed using flow cytometry ( Fig. 3g ). These data suggested that cAMP amplifies IFN-γ and IL-2 signalling in T cells through the upregulation of IFN-γR1 and IL-2Rβ, respectively. 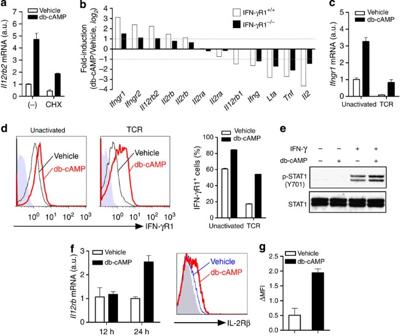Figure 3: cAMP amplifies IFN-γ and IL-2 signalling through induction of IFN-γR1 and IL-2Rβ. (a) Expression ofIl12rb2mRNA in T cells activated with αCD3/CD28 for 24 h with addition of db-cAMP or cycloheximide (CHX) or both for the last 12 h. (b) Profile of db-cAMP-dependent expression of cytokines and their receptors by WT or IFN-γR1−/−T cells activated for 12 h with αCD3/CD28 followed by treatment with db-cAMP or vehicle for another 3 h. Data shown in bar graphs represents fold change (db-cAMP versus vehicle) in mean intensity from each probe in biological duplicates. The probe forIfngr1in this array is targeted to a segment of sequence in the exon VII, while The IFN-γR1−/−mouse that we used hasIfngr1gene disrupted by inserting the neomycin resistance gene into exon V. (c,d) Expression of IFN-γR1 mRNA (c) and protein (d) in T cells stimulated with or without αCD3/CD28 in the absence or presence of db-cAMP for 12 h. (e) Immunoblot for p-STAT1 (Y701) and STAT1 in T cells pretreated with db-cAMP for 12 h, washed and restimulated with 1 ng ml−1IFN-γ for another 30 min. (f) Expression ofIl2rbmRNA in T cells treated with db-cAMP for 12 and 24 h. (g) IL-2Rβ protein expression in T cells activated with αCD3/CD28 for 2 days, allowed to rest for another 2 days, then restimulated with db-cAMP in the presence of IL-2 for 24 h. Data shown as mean±s.e.m. are representative of two independent experiments with triplicates (a,c–g) or are from one experiment (b). a.u., arbitrary units. Figure 3: cAMP amplifies IFN-γ and IL-2 signalling through induction of IFN-γR1 and IL-2Rβ. ( a ) Expression of Il12rb2 mRNA in T cells activated with αCD3/CD28 for 24 h with addition of db-cAMP or cycloheximide (CHX) or both for the last 12 h. ( b ) Profile of db-cAMP-dependent expression of cytokines and their receptors by WT or IFN-γR1 −/− T cells activated for 12 h with αCD3/CD28 followed by treatment with db-cAMP or vehicle for another 3 h. Data shown in bar graphs represents fold change (db-cAMP versus vehicle) in mean intensity from each probe in biological duplicates. The probe for Ifngr1 in this array is targeted to a segment of sequence in the exon VII, while The IFN-γR1 −/− mouse that we used has Ifngr1 gene disrupted by inserting the neomycin resistance gene into exon V. ( c , d ) Expression of IFN-γR1 mRNA ( c ) and protein ( d ) in T cells stimulated with or without αCD3/CD28 in the absence or presence of db-cAMP for 12 h. ( e ) Immunoblot for p-STAT1 (Y701) and STAT1 in T cells pretreated with db-cAMP for 12 h, washed and restimulated with 1 ng ml −1 IFN-γ for another 30 min. ( f ) Expression of Il2rb mRNA in T cells treated with db-cAMP for 12 and 24 h. ( g ) IL-2Rβ protein expression in T cells activated with αCD3/CD28 for 2 days, allowed to rest for another 2 days, then restimulated with db-cAMP in the presence of IL-2 for 24 h. Data shown as mean±s.e.m. are representative of two independent experiments with triplicates ( a , c – g ) or are from one experiment ( b ). a.u., arbitrary units. Full size image Requirement of CREB for cAMP-induced IL-12Rβ2 and IFN-γR1 We next investigated the molecular mechanisms of how cAMP directly induces IL-12Rβ2 and IFN-γR1 expression. The db-cAMP-induced Il12rb2 and Ifngr1 expression was mimicked by a PKA-specific agonist N 6 -Bnz-cAMP (ref. 34 ) ( Fig. 4a ) and attenuated by PKA inhibitors ( Fig. 4b ) in unactivated T cells, which produced neither IL-2 nor IFN-γ. We transfected unactivated T cells with a small interfering RNA (siRNA) for Creb1 or a scrambled siRNA and then stimulated T cells with db-cAMP. Creb1 -specific siRNA reduced CREB expression in transfected cells ( Fig. 4c ) and suppressed cAMP-induced Il12rb2 and Ifngr1 expression compared with those in T cells transfected with scrambled siRNA ( Fig. 4d ). CREB is usually activated by phosphorylation at Ser133, p-CREB(S133), which promotes transcription by recruitment of the coactivator CREB-binding protein to gene loci [17] . However, although TCR or phorbol-12-myristate-13-acetate (PMA) plus ionomycin could induce CREB activation ( Fig. 4e ), they did not induce, but rather reduced Il12rb2 or Ifngr1 expression under the condition where cAMP induced both mRNAs ( Fig. 4f ). These results suggest requirement of other factors downstream of PKA in addition to p-CREB(S133). 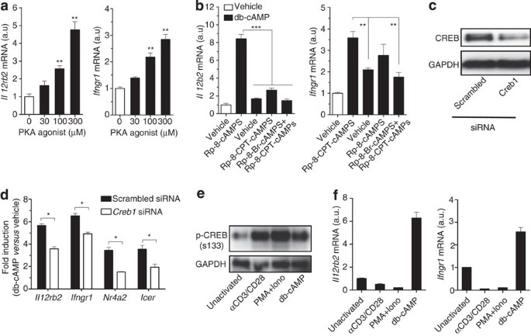Figure 4: Activation of PKA-CREB pathway is required but insufficient for cAMP-induced IL-12Rβ2 and IFN-γR1 expression. (a) Expression ofIl12rb2andIfngr1mRNA in T cells stimulated with indicated concentrations of a PKA agonist, N6-Bnz-cAMP, for 12 h. (b) Expression ofIl12rb2andIfngr1mRNA in T cells stimulated with db-cAMP in the presence of PKA inhibitor, Rp-8-Br-cAMPS and/or Rp-8-CPT-cAMPS for 12 h. (c,d) T cells treated with scrambled orCreb1siRNA for 48 h, followed by immunoblot for CREB (c) or stimulated with db-cAMP for another 12 h for detection of mRNA expression (d). mRNA expression is normalized to vehicle-treated of each siRNA-transfected cells.IcerandNr4a2were used as positive controls for CREB-dependent genes. (e) Immunoblot for p-CREB(S133) in IFN-γR1−/−T cells stimulated without (unactivated) or with either αCD3/CD28, PMA (20 ng ml−1) plus ionomycin (500 ng ml−1) (PMA+Iono), or db-cAMP for 30 min. (f) Expression ofIl12rb2andIfngr1mRNA in IFN-γR1−/−T cells stimulated as inein the presence of anti-IL-2 for 12 h. Data shown as mean±s.e.m. are representative of two (a–c,e,f) or four (d) independent experiments with triplicates. Statistical significance was examined by unpaired two-tailed student’st-test, *P<0.05; **P<0.01; ***P<0.001. a.u., arbitrary units. Figure 4: Activation of PKA-CREB pathway is required but insufficient for cAMP-induced IL-12Rβ2 and IFN-γR1 expression. ( a ) Expression of Il12rb2 and Ifngr1 mRNA in T cells stimulated with indicated concentrations of a PKA agonist, N 6 -Bnz-cAMP, for 12 h. ( b ) Expression of Il12rb2 and Ifngr1 mRNA in T cells stimulated with db-cAMP in the presence of PKA inhibitor, Rp-8-Br-cAMPS and/or Rp-8-CPT-cAMPS for 12 h. ( c , d ) T cells treated with scrambled or Creb1 siRNA for 48 h, followed by immunoblot for CREB ( c ) or stimulated with db-cAMP for another 12 h for detection of mRNA expression ( d ). mRNA expression is normalized to vehicle-treated of each siRNA-transfected cells. Icer and Nr4a2 were used as positive controls for CREB-dependent genes. ( e ) Immunoblot for p-CREB(S133) in IFN-γR1 −/− T cells stimulated without (unactivated) or with either αCD3/CD28, PMA (20 ng ml −1 ) plus ionomycin (500 ng ml −1 ) (PMA+Iono), or db-cAMP for 30 min. ( f ) Expression of Il12rb2 and Ifngr1 mRNA in IFN-γR1 −/− T cells stimulated as in e in the presence of anti-IL-2 for 12 h. Data shown as mean±s.e.m. are representative of two ( a – c , e , f ) or four ( d ) independent experiments with triplicates. Statistical significance was examined by unpaired two-tailed student’s t -test, * P <0.05; ** P <0.01; *** P <0.001. a.u., arbitrary units. Full size image Involvement of CRTC2 in cAMP-induced IL-12Rβ2 and IFN-γR1 One candidate for such factors is CRTC2 that is regulated negatively by SIK2 and functions as a CREB coactivator in many types of cells [19] , [20] , [21] , [22] . Stimulation of T cells with db-cAMP induced not only phosphorylation of CREB but also dephosphorylation of CRTC2 ( Fig. 5a ), decreased the amount of CRTC2 in the cytoplasm and increased the amount of dephosphorylated CRTC2 in the nucleus ( Fig. 5b ). This distribution is SIK-dependent, because SIK2 –/– T cells [22] constitutively showed more nuclear CRTC2 than WT cells, which increased little by cAMP ( Fig. 5c ). As reported [18] , [19] , protein kinase inhibitor staurosporine (STS) induced dephosphorylation and nuclear translocation of CRTC2 without enhancing CREB phosphorylation ( Fig. 5b ). To investigate whether cAMP affects transcriptional activity of CRTC2, we performed a reporter assay with GAL4-fusion CRTC2 in WT and SIK2 –/– T cells. While db-cAMP increased GAL4-transcriptional activity in WT cells, the basal GAL4 activity was already higher in SIK2 –/– T cells and no further increase was observed upon cAMP addition ( Fig. 5d ). These findings suggest that SIK2-CRTC2 pathway functions downstream of cAMP in T cells. 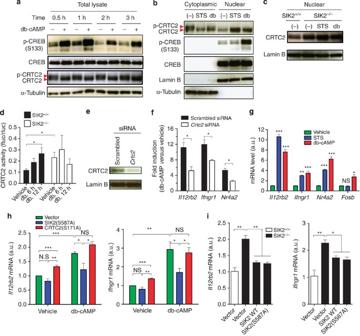Figure 5: SIK2-CRTC2 signalling mediates cAMP-induced expression ofIl12rb2andIfngr1. (a) cAMP induces CREB phosphorylation and CRTC2 dephosphorylation in T cells. (b) cAMP and STS reduces cytoplasmic CRTC2 and increases nuclear CRTC2 in T cells that were rested for 2 days and then stimulated for 1 h. (c) cAMP does not increase nuclear CRTC2 in SIK2−/−T cells. (d) GAL4 reporter assay of CRTC2 activity of SIK2+/+or SIK2−/−T cells that were transfected with GAL4-fusion pM-mCRTC2 and pTAL-5xGAL4-Luciferase reporter and stimulated with db-cAMP for the indicated times. The activity is shown as the ratio of firefly luciferase activity to renilla pRL-TK luciferase activity. (e,f) T cells were transfected with scrambled orCrtc2siRNA for 36 h, followed by immunobloting of CRTC2 (e) or stimulating with db-cAMP for another 12 h for detection of mRNA expression (f). mRNA expression in db-cAMP-treated cells is normalized to vehicle-treated of each siRNA-transfected cells. (g) Expression of indicated mRNA in T cells stimulated with STS or db-cAMP for 12 h. (h) CRTC2(S171A) increases basal expression ofIl12rb2andIfngr1, while SIK2(S587A) reduces cAMP-induced expression of these genes in TCR-activated T cells. (i) SIK2 WT and S587A mutant reduce basal expression ofIl12rb2andIfngr1in SIK2-deficient T cells. Data shown as mean±s.e.m. are representative of two (a–e,i) or three (f,g) independent experiments with triplicates or are from four independent experiments (h). Statistical significance was examined by unpaired two-tailed student’st-test, *P<0.05; **P<0.01; ***P<0.001. NS, not significant; a.u., arbitrary units. Figure 5: SIK2-CRTC2 signalling mediates cAMP-induced expression of Il12rb2 and Ifngr1. ( a ) cAMP induces CREB phosphorylation and CRTC2 dephosphorylation in T cells. ( b ) cAMP and STS reduces cytoplasmic CRTC2 and increases nuclear CRTC2 in T cells that were rested for 2 days and then stimulated for 1 h. ( c ) cAMP does not increase nuclear CRTC2 in SIK2 −/− T cells. ( d ) GAL4 reporter assay of CRTC2 activity of SIK2 +/+ or SIK2 −/− T cells that were transfected with GAL4-fusion pM-mCRTC2 and pTAL-5xGAL4-Luciferase reporter and stimulated with db-cAMP for the indicated times. The activity is shown as the ratio of firefly luciferase activity to renilla pRL-TK luciferase activity. ( e , f ) T cells were transfected with scrambled or Crtc2 siRNA for 36 h, followed by immunobloting of CRTC2 ( e ) or stimulating with db-cAMP for another 12 h for detection of mRNA expression ( f ). mRNA expression in db-cAMP-treated cells is normalized to vehicle-treated of each siRNA-transfected cells. ( g ) Expression of indicated mRNA in T cells stimulated with STS or db-cAMP for 12 h. ( h ) CRTC2(S171A) increases basal expression of Il12rb2 and Ifngr1 , while SIK2(S587A) reduces cAMP-induced expression of these genes in TCR-activated T cells. ( i ) SIK2 WT and S587A mutant reduce basal expression of Il12rb2 and Ifngr1 in SIK2-deficient T cells. Data shown as mean±s.e.m. are representative of two ( a – e , i ) or three ( f , g ) independent experiments with triplicates or are from four independent experiments ( h ). Statistical significance was examined by unpaired two-tailed student’s t -test, * P <0.05; ** P <0.01; *** P <0.001. NS, not significant; a.u., arbitrary units. Full size image To corroborate that SIK2-CRTC2 pathway mediates cAMP-induced expression of Il12rb2 and Ifngr1 , we depleted CRTC2 in T cells by siRNA ( Fig. 5e ). CRTC2 depletion considerably suppressed db-cAMP-induced Il12rb2 and Ifngr1 expression ( Fig. 5f ). Conversely, STS induced expression of Il12rb2 and Ifngr1 mRNA as potently as db-cAMP ( Fig. 5g ). Expression of Nr4a2 , a gene known to be regulated by CRTC2 and p-CREB [35] , was also reduced by CRTC2 siRNA and induced by STS and db-cAMP ( Fig. 5f ), while another p-CREB-target gene Fosb was induced only by db-cAMP ( Fig. 5g ), probably reflecting less CRTC2 contribution [35] . Consistently, overexpression of a constitutively active form of CRTC2, CRTC2(S171A), which could not be phosphorylated at the site Ser171 and, therefore, retained in the nucleus [20] , enhanced the basal expression of Il12rb2 and Ifngr1 , while overexpression of a constitutively active form of SIK2, SIK2(S587A), which constitutively phosphorylated CRTC2 and thus prevented CRTC2 nuclear translocation [36] , suppressed the db-cAMP-induced Il12rb2 and Ifngr1 expression ( Fig. 5h ). Furthermore, comparing to WT cells, SIK2 –/– T cells have a higher level of Il12rb2 and Ifngr1 mRNA, which could be suppressed by overexpression of WT SIK2 or the SIK2(S587A) mutant ( Fig. 5i ). These data suggest that CRTC2 mediates cAMP-PKA signalling-induced expression of Il12rb2 and Ifngr1 . Binding of p-CREB and CRTC2 to Il12rb2 and Ifngr1 gene loci Computational analysis identified several putative half or full CRE sites in the promoter/enhancer regions of Il12rb2 and Ifngr1 gene loci ( Fig. 6a ). We performed chromatin immunoprecipitation analysis and observed that upon cAMP stimulation, p-CREB(S133) and CRTC2 were recruited to several of these sites located from −3.6 to +0.8 kb in Il12rb2 gene locus ( Fig. 6b , sites E–L). Similarly, cAMP increased binding of p-CREB(S133) and CRTC2 to two sites around the transcription start site and one site at position +4.6 kb in the first intron of Ifngr1 gene ( Fig. 6c , sites M, N and P). These results suggest that CREB and CRTC2 activated by cAMP are recruited to the sites in the promoter/enhancer regions of Il12rb2 or Ifngr1 gene loci. 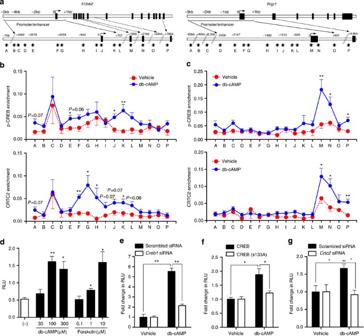Figure 6: Recruitment of p-CREB and CRTC2 toIl12rb2andIfngr1gene loci upon cAMP stimulation. (a) Schematic diagram of the mouseIl12rb2(left) andIfngr1(right) genes and their promoter/enhancer regions illustrating potential CRE sites and the positions of the primers. (b,c) Enrichment of p-CREB(S133) (upper) and CRTC2 (lower) at theIl12rb2(b) andIfngr1(c) gene loci. T cells were rested for 2 days followed by stimulation with db-cAMP or vehicle for 1 h. Cells were fixed, and chromatin immunoprecipitation was performed using anti-p-CREB (S133) and anti-CRTC2. Data are normalized to the input DNA and represent eight individual chromatin immunoprecipitations from four independent experiments (mean±s.e.m.). (d–g) Luciferase activity of EL4 cells stably expressing theIl12rb2luciferase reporter, stimulated for 24 h with indicated concentrations of db-cAMP, forskolin or vehicle (d), or stimulated for 24 h with db-cAMP after 40 h treatment with scrambled orCreb1siRNA (e), after 24 h transfection with WT CREB or the CREB(S133A) mutant (f) or after 40 h treatment with scrambled orCrtc2siRNA (g). Relative light unit (RLU) is normalized to vehicle control of each transfection condition (e–g). Data shown as mean±s.e.m. are representative of two (d–g) independent experiments with triplicates. Statistical significance was examined by unpaired two-tailed Student’st-test, *P<0.05; **P<0.01. Figure 6: Recruitment of p-CREB and CRTC2 to Il12rb2 and Ifngr1 gene loci upon cAMP stimulation. ( a ) Schematic diagram of the mouse Il12rb2 (left) and Ifngr1 (right) genes and their promoter/enhancer regions illustrating potential CRE sites and the positions of the primers. ( b , c ) Enrichment of p-CREB(S133) (upper) and CRTC2 (lower) at the Il12rb2 ( b ) and Ifngr1 ( c ) gene loci. T cells were rested for 2 days followed by stimulation with db-cAMP or vehicle for 1 h. Cells were fixed, and chromatin immunoprecipitation was performed using anti-p-CREB (S133) and anti-CRTC2. Data are normalized to the input DNA and represent eight individual chromatin immunoprecipitations from four independent experiments (mean±s.e.m.). ( d – g ) Luciferase activity of EL4 cells stably expressing the Il12rb2 luciferase reporter, stimulated for 24 h with indicated concentrations of db-cAMP, forskolin or vehicle ( d ), or stimulated for 24 h with db-cAMP after 40 h treatment with scrambled or Creb1 siRNA ( e ), after 24 h transfection with WT CREB or the CREB(S133A) mutant ( f ) or after 40 h treatment with scrambled or Crtc2 siRNA ( g ). Relative light unit (RLU) is normalized to vehicle control of each transfection condition ( e – g ). Data shown as mean±s.e.m. are representative of two ( d – g ) independent experiments with triplicates. Statistical significance was examined by unpaired two-tailed Student’s t -test, * P <0.05; ** P <0.01. Full size image We cloned a −4.6 kb to +70 bp fragment of the Il12rb2 promoter/enhancer region in the pGL4 luciferase reporter vector, transfected it into EL4 cells and stimulated with db-cAMP or forskolin. db-cAMP and forskolin induced Il12rb2 promoter reporter activity ( Fig. 6d ) and this cAMP-induced Il12rb2 promoter activity was suppressed by treatment with Creb1 siRNA, overexpression of the CREB(S133A) mutant or Crtc2 siRNA ( Fig. 6e–g ), indicating that both p-CREB(S133) and CRTC2 regulate cAMP-activated Il12rb2 transcription. EP4 signalling in T cells enhances Th1 inflammation in vivo To study whether PGE 2 -EP4-cAMP signalling in T cells regulates cytokine receptors and Th1 response in vivo , we generated mice with deletion of EP4 in T cells by crossing Lck-Cre mice [37] with EP4-floxed mice [38] . Loss of EP4 in CD4 + T cells was confirmed in Lck-Cre + EP4 fl/+ and Lck-Cre + EP4 fl/fl mice ( Fig. 7a ). To investigate whether EP4 deficiency in T cells affects in vivo Th1 differentiation and expression of Th1-related cytokine receptors, we used the CHS model and immunized Lck-Cre − EP4 fl/fl or Lck-Cre + EP4 fl/fl mice by painting the shaved abdomen with dinitrofluorobenzene (DNFB) on day 0 and purified CD4 + T cells in draining lymph nodes (dLNs) on day 5. CD4 + T cells from Lck-Cre + EP4 fl/fl mice produced less amounts of IFN-γ and IL-2 ( Fig. 7b ) and exhibited less mRNA expression of Th1 cytokine receptors, for example, Il12rb2 , Ifngr1 , Il2rb and CREB/CRTC2-targeted gene Icer than T cells from littermate control Lck-Cre − EP4 fl/fl mice ( Fig. 7c ). Consistent with the above results, the numbers of IL-12Rβ2- and IFN-γR1-expressing CD4 + T cells in dLNs from Lck-Cre + EP4 fl/fl mice were also lower than those from control mice ( Fig. 7d ). We also found that Cd69 gene expression and the number of CD4 + CD69 + T cells were decreased in dLNs from DNFB-sensitized Lck-Cre + EP4 fl/fl mice ( Fig. 7c ). Moreover, when we adoptively transferred dLN cells from DNFB-sensitized Lck-Cre + EP4 fl/fl or Lck-Cre − EP4 fl/fl mice into naive C57BL/6 mice on day 5 and immediately challenged the recipient mice by painting the same antigen on the ear, transfer of EP4-deficient T cells induced less ear swelling ( Fig. 7e ). 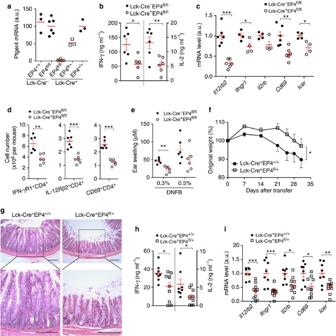Figure 7: EP4-cAMP signalling in T cells modulates expression of IL-12Rβ2 and IFN-γR1, and Th1 responsein vivo. (a) Expression ofPtger4mRNA in CD4+T cells of mice of indicated genotypes. (b) IFN-γ and IL-2 production by dLN CD4+T cells isolated from DNFB-sensitized mice on day 5 and then stimulated with αCD3/CD28 for 24 h. (c) mRNA expression of Th1-related cytokine receptor genes in dLN CD4+T cells isolated from DNFB-sensitized mice on day 5.Il12rb2andCd69mRNA are shown in dLN CD4+T cells stimulated with αCD3/CD28 for 24 h. (d) Numbers of IL-12Rβ2-, IFN-γR1-, or CD69-positive CD4+T cells in dLNs of DNFB-sensitized mice on day 5. (e) Ear swelling of WT recipient mice given intravenous transfer of dLN cells from DNFB-sensitized Lck-Cre−EP4fl/flor Lck-Cre+EP4fl/flmice. (f) Change in body weight ofRag2−/−mice (8–10 mice per group) given intravenous transfer of Lck-Cre+EP4+/+or Lck-Cre+EP4fl/+naive T cells. (g) Hematoxylin and eosin staining of the colon ofRag2−/−mice 42 days after transfer. Scale bar, 200 μM. (h,i) IFN-γ and IL-2 production (h) and mRNA expression of indicated genes (i) in CD4+T cells isolated from the mLNs ofRag2–/–mice 42 days after transfer and stimulated with αCD3 for 3 days. Horizontal and error bars represent the mean and s.e.m., respectively. Statistical significance inewas examined by two-way ANOVA. *P<0.05; **P<0.01; ***P<0.001. a.u., arbitrary units. Figure 7: EP4-cAMP signalling in T cells modulates expression of IL-12Rβ2 and IFN-γR1, and Th1 response in vivo. ( a ) Expression of Ptger4 mRNA in CD4 + T cells of mice of indicated genotypes. ( b ) IFN-γ and IL-2 production by dLN CD4 + T cells isolated from DNFB-sensitized mice on day 5 and then stimulated with αCD3/CD28 for 24 h. ( c ) mRNA expression of Th1-related cytokine receptor genes in dLN CD4 + T cells isolated from DNFB-sensitized mice on day 5. Il12rb2 and Cd69 mRNA are shown in dLN CD4 + T cells stimulated with αCD3/CD28 for 24 h. ( d ) Numbers of IL-12Rβ2-, IFN-γR1-, or CD69-positive CD4 + T cells in dLNs of DNFB-sensitized mice on day 5. ( e ) Ear swelling of WT recipient mice given intravenous transfer of dLN cells from DNFB-sensitized Lck-Cre − EP4 fl/fl or Lck-Cre + EP4 fl/fl mice. ( f ) Change in body weight of Rag2 −/− mice (8–10 mice per group) given intravenous transfer of Lck-Cre + EP4 +/+ or Lck-Cre + EP4 fl/+ naive T cells. ( g ) Hematoxylin and eosin staining of the colon of Rag2 −/− mice 42 days after transfer. Scale bar, 200 μM. ( h , i ) IFN-γ and IL-2 production ( h ) and mRNA expression of indicated genes ( i ) in CD4 + T cells isolated from the mLNs of Rag2 –/– mice 42 days after transfer and stimulated with αCD3 for 3 days. Horizontal and error bars represent the mean and s.e.m., respectively. Statistical significance in e was examined by two-way ANOVA. * P <0.05; ** P <0.01; *** P <0.001. a.u., arbitrary units. Full size image We next isolated CD45RB hi CD25 − CD4 + naive T cells from the spleen of Lck-Cre + EP4 +/+ or Lck-Cre + EP4 fl/+ mice, transferred them into mice deficient in recombination-activating gene 2 ( Rag2 –/– mice), and monitored development and progression of colitis. Transfer of naive T cells of both genotypes induced colitis in Rag2 –/– mice. However, the transfer of Lck-Cre + EP4 fl/+ T cells induced milder body weight loss ( Fig. 7f ) and weaker colonic inflammation than that of T cells from littermate control Lck-Cre + EP4 +/+ mice ( Fig. 7g ). Moreover, mesenteric lymph node CD4 + T cells from Rag2 –/– mice reconstituted with Lck-Cre + EP4 fl/+ T cells produced less amounts of IFN-γ and IL-2 ( Fig. 7h ) and expressed lower levels of Il12rb2 , Ifngr1 , Il2rb, Cd69 and Icer mRNA ( Fig. 7i ) than CD4 + T cells from Rag2 –/– mice reconstituted with Lck-Cre + EP4 +/+ T cells. We also repeated this transfer experiment using CD45RB hi CD25 − CD4 + naive T cells from Lck-Cre + EP4 fl/fl mice or EP2 −/− mice. We have found attenuation of the colitis also in the Rag2 −/− mice reconstituted with Lck-Cre + EP4 fl/fl T cells and have not found any difference of colitis development between the groups of mice that received WT and EP2 −/− T cells (data not shown). These results confirm the importance of EP4 and indicate that EP2 has, if any, a minor role in T cells, a loss of which can be compensated for by EP4. Here we have dissected the molecular mechanism underlying PGE 2 -induced facilitation of Th1 differentiation, and revealed the role of cAMP in this process. PGE 2 acts on EP2 or EP4 receptors to generate cAMP and cAMP activates PKA, which in turn directly phosphorylates CREB and induces dephosphorylation and nuclear translocation of CRTC2 through inhibiting SIK2. Activated CREB and CRTC2 together promote gene transcription of IL-12Rβ2 and IFN-γR1, receptors for two critical cytokines of Th1 differentiation. Our findings are consistent with recent reports that PGI 2 -IP signalling promotes Th1 differentiation through cAMP-PKA pathway in vitro and enhances CHS responses in vivo [39] , and that Gαs-deficient T cells which fail to produce cAMP, show impaired differentiation into Th1 cells and that the addition of cAMP analogue restores Th1 differentiation in these cells [16] . Our study has thus verified the facilitative role of cAMP in Th1 differentiation by clarifying its molecular mechanism. A question remains as to how these findings are reconciled with the long-held, traditional view that cAMP suppresses Th1 differentiation [8] . Here we found that cAMP-mediated inhibition of TCR-induced expression of CD25, production of IL-2 and IFN-γ, Th1 differentiation and cell proliferation could all be rescued or even overcome by strengthening CD28 costimulation in a PI3K-dependent manner. Simultaneous activation of PI3K at cAMP generation by PGE 2 -EP2/EP4 signalling [9] combined with that by CD28 costimulation can cancel out the cAMP-mediated inhibition of TCR signalling, and preserve, for example, expression of critical genes such as CD25, IL-2 and IFN-γ. The primary inhibitory site by cAMP may be Lck. Tasken and his collaborators suggested that PKA interferes with LCK activation, and this action can be antagonized by PI3K activation following CD28 costimulation [33] , [40] . Then, how important is this PGE 2 -cAMP-dependent mechanism in Th1-mediated immune response in vivo and in human immune diseases? Here we have used two disease models and demonstrated that EP4-cAMP signalling in T cells facilitated expression of Th1 cytokine receptors and Th1 response in vivo . We have generated mice with selective deletion of EP4 in T cells, and revealed that the loss of EP4 in T cells considerably attenuates CHS response and the adoptive transfer colitis. In both models, selective blockade of EP4 in T cells prevented in vivo Th1 differentiation with downregulated expression of Il12rb2 , Ifngr1 and Il2rb genes and other CREB/CRTC2-dependent genes in lymph nodes (LNs) CD4 + T cells. CHS is a mouse model of allergic contact dermatitis in humans, in which IFN-γ produced by CD4 + Th1 and CD8 + type 1 cytotoxic T cells has an important role [41] . The adoptive transfer colitis is a model of inflammatory bowel disease, particularly CD [42] . Genome-wide association studies have revealed that the PTGER4 , IL12RB2 and IL2RA (human IL-2Rα) genes are linked to risk loci associated with CD [13] , [14] . High expression of IL12RB2 , IL2RA and IL2RB (encoding human IL-2Rβ) genes was found in blood or in lamina propria CD4 + T cells of patients with CD [43] , [44] . Upregulation of CREB was also found in peripheral blood mononuclear cells from patients with inflammatory diseases including CD [45] . Additionally, in experimental allergic encephalomyelitis, a mouse model for multiple sclerosis, systemic inhibition of EP4 suppressed Th1 differentiation and IFN-γ production [9] , [46] . Interestingly, PTGER4 and IL12RB2 were shown to be associated with multiple sclerosis [12] , [15] . Thus, our results showed that EP4-cAMP signalling in T cells has a critical role in regulation of cytokine signalling and Th1 response in vivo using various mouse models of immune inflammation and suggest the possibility of similar actions operating clinically in human diseases. Here we have demonstrated how cAMP signalling facilitates Th1 differentiation, and shown that PGE 2 -EP4 signalling is representative of such cAMP signalling operating in T cells. 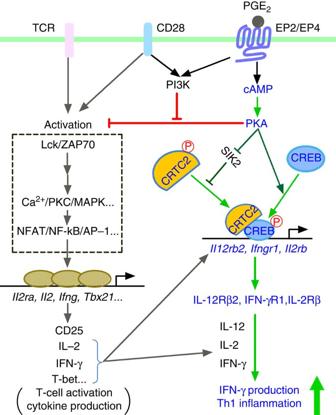Figure 8: A model for synergistic action of cAMP and PI3K in Th1 differentiation. cAMP generated in response to PGE2binding to EP2/EP4 activates PKA, which phosphorylates CREB and activates CRTC2 through phosphorylation of SIK. Activated CREB and CRTC2 translocate to the nucleus and induce expression ofIl12rb2, Ifngr1and possiblyIl2rb, thus facilitating Th1 differentiation synergistically with IL-12, IFN-γ and IL-2. While cAMP-PKA inhibits T-cell activation by suppressing TCR signalling, coactivation of PI3K by EP2/EP4 and CD28 cancels this inhibition and promotes the Th1-facilitative action of cAMP. Figure 8 depicts our model for cAMP-mediated Th1 differentiation and its cross-talk with PI3K pathway in TCR activation. In addition to prostanoids, there are a number of other agents that can activate cAMP signalling in T cells, such as catecholamines, histamine and adenosine [8] . Our results suggest a possibility that these substances similarly facilitate Th1 differentiation and promote immune inflammation. This is particularly the case for those substances that activates both PI3K and cAMP signalling simultaneously. Given that most of these receptors are G-protein coupled receptors (GPCRs), our present results show how GPCR signalling cooperates with cytokine signalling, that is, amplifying the latter actions by inducing their receptors. We propose to designate such GPCR actions as cytokine amplification and ligands of such GPCR as cytokine amplifiers. This cytokine amplifying action of GPCR ligands surely accounts for some of their pathophysiological actions and may, therefore, be of therapeutic consideration. Figure 8: A model for synergistic action of cAMP and PI3K in Th1 differentiation. cAMP generated in response to PGE 2 binding to EP2/EP4 activates PKA, which phosphorylates CREB and activates CRTC2 through phosphorylation of SIK. Activated CREB and CRTC2 translocate to the nucleus and induce expression of Il12rb2, Ifngr1 and possibly Il2rb , thus facilitating Th1 differentiation synergistically with IL-12, IFN-γ and IL-2. While cAMP-PKA inhibits T-cell activation by suppressing TCR signalling, coactivation of PI3K by EP2/EP4 and CD28 cancels this inhibition and promotes the Th1-facilitative action of cAMP. Full size image Mice C57BL/6 mice were obtained from Japan SLC (Shizuoka, Japan). EP2- and EP4-deficient and littermate control WT mice have been previously described [9] . Mice defective in IFN-γR1 on a C57BL/6 background [30] were kind gifts from M. Aguet. To generate EP4-deficient T cells, Lck-Cre mice [37] were crossed to lox-flanked Ptger4 mice [38] . SIK2 −/− mice have been described elsewhere [22] and were housed in the National Institute of Biomedical Innovation. All mice, except the SIK2 −/− mice, were housed at the Institute of Laboratory Animals of Kyoto University on a 12-h light/dark cycle under specific pathogen-free conditions. All experimental procedures were approved by the Committee on Animal Research of Kyoto University Faculty of Medicine and National Institute of Biomedical Innovation. Plasmids WT CREB and the CREB(S133A) mutant plasmids were kindly provided by H. Bito. pGFP-mSIK2, pGFP-mSIK2 S587A, pGFP-mCRTC2 S171A and GAL4 fused pM-mCRTC2 and pTAL-5x GAL4 have been described [16] , [34] . Reagents PGE 2 (100 nM) was obtained from Cayman Chemical. Agonists selective to each EP subtype (ONO-DI-004, ONO-AE1-259, ONO-AE-248 and ONO-AE1-329 for EP1, EP2, EP3 and EP4, respectively, each 100 nM) were kind gifts of Ono Pharmaceutical Co., Japan. Dibutyryl cAMP (db-cAMP, 100 μM), N 6 -Bnz-cAMP (30–300 μM), wortmannin (100 nM), LY-294002 (1 μM), H-89 (10 μM), Rp-8-CPT-cAMPS (300 μM), Rp-8-Br-cAMPS (300 μM), Forskolin (1 μM) and 3-isobutyl-1-methylxanthine (100 μM) were purchased from Sigma. Cycloheximide (10 μM) and STS (5–50 nM) were purchased from Calbiochem. Preparation and culture of CD4 + T cells Naive CD4 + CD45RB + CD25 − and CD4 + T cells were purified from spleens and LNs by using FACS Aria2 (Becton Dickinson) and auto-MACS (Miltenyi), respectively. Cells were cultured in complete RPMI1640 medium containing 10% FBS. For in vitro activation of T cells, plate-bound antibodies to CD3 (10 μg ml −1 , clone 145-2C11, eBioscience) and CD28 (10 μg ml −1 or indicated concentrations, clone 37.51, eBioscience) were used. For T H 1 differentiation, cells were stimulated with anti-CD3 and anti-CD28 for the first 2 days, and then without anti-CD3 and anti-CD28 antibodies for another 24 h. Cells were cultured with 2,500 U ml −1 rmIL-2, 10 ng ml −1 rmIL-12 (R&D Systems) and 5 μg ml −1 anti-IL-4 (clone 11B11, eBioscience) for 3 days. To reduce the background of phosphorylated CREB, freshly isolated CD4 + T cells were cultured for 2 days in RPMI1640 medium and IL-7 (10 ng ml −1 , R&D Systems) that was added to maintain the survival of naive T cells [47] . In some culture conditions, 10 ng ml −1 of IFN-γ (R&D Systems) or 10 μg ml −1 of anti-mouse IFN-γ (clone XMG1.2, eBioscience), anti-mouse IL-12/IL-23 p40 (clone C17.8, eBioscience) or anti-mouse IL-2 (clone JES6-1A12, eBioscience) were added. Surface and intracellular staining For surface staining, CD4 + T cells were directly stained with phycoerythrin (PE)-conjugated anti-mouse CD119 (IFN-γR1, clone 2E2, eBioscience), PE-conjugated rat anti-mouse CD122 (IL-2Rβ, clone TM-β1, BD Pharmingen) or PE-conjugated anti-mouse CD69 (clone H1.2F3, eBioscience), or stained firstly with hamster anti-mouse IL-12Rβ2 (BD Pharmingen) and then with PE-conjugated mouse anti-Armenian and Syrian hamster IgG cocktail (BD Pharmingen). For intracellular staining, CD4 + T cells were restimulated with 50 ng ml −1 PMA (Sigma) and 500 ng ml −1 ionomycin (Sigma) in the presence of GolgiPlug (BD Pharmingen) for the last 4–5 h of incubation. Cells were fixed and permeabilized with Cytofix/Cytoperm (BD Pharmingen) and stained with fluorescein isothiocyanate (FITC)-conjugated antibody to IFN-γ (clone XMG1.2, eBioscience), and PE-conjugated antibody to IL-4 (clone 11B11, eBioscience). Quantitative flow cytometry was performed on an Epics XL-MCL (Beckman Coulter) or FACS Calibur (BD Bioscience). Fractionation and western blot Cytoplasmic and nuclear cell fractions were prepared using ProteoExtract Subcellular Proteome Extraction kit (Calbiochem). Western blotting was performed according to a protocol from Cell Signaling. Anti-mouse CREB, p-CREB (S133), STAT1, and p-STAT1 (Y701) antibodies were obtained from Cell Signaling. Anti-mouse GAPDH (6C5, Ambion), anti-mouse α-tubulin (DM 1A, Sigma) and anti-goat lamin B (C-20, Santa Cruz) were used as internal control. Anti-rabbit CRTC2 anti-serum has been described [20] . Immunoreactive proteins were visualized by using the enhanced chemiluminescence system from Fuji Film (LAS-3000). Enzyme-linked immunosorbent assay For the detection of IL-2 and IFNγ production, the supernatants of cell cultures were collected, and the manufacturer’s instructions were followed (Pierce). Real-time PCR RNA purification and reverse transcription were performed by using Rneasy Mini Kit (Qiagen) and High-capacity cDNA Reverse Transcription Kits (ABI), respectively. Samples were analysed by real-time PCR with FastStart DNA Master PLUS SYBR Green I kit or LightCycler Taqman Master kit with Universal ProbeLibrary Set, Mouse (Roche). Primers and probes used in this study are listed in Supplementary Table S1 . Expression was normalized to that of mouse 18S ribosomal RNA ( Rn18s ) or glyceraldehyde-3-phosphate dehydrogenase ( Gapdh ) gene and calculated relative to expression in vehicle control by the 2 –ΔΔCt method in each experiment. Microarray assay mRNA was converted to biotinylated antisense RNA using GeneChip HT 3′IVT Express Kit (Affymetrix) and biological duplicates were hybridized to Affymetrix GenChip Mouse Genome 430 2.0 Arrays (Affymetrix). Data were scaled, normalized by GeneChip Operating Software 1.4. After filtration, expression levels of selected probes were shown in bar graphs by using mean intensity of biological duplicates. Microarray data were deposited in GEO Data Sets under accession number GSE39592 . Chromatin immunoprecipitation Freshly isolated WT CD4 + T cells were cultured for 2 days in the presence of IL-7 followed by stimulation with db-cAMP (100 μM) or vehicle for another 1 h. Cells were crosslinked with 1% (vol/vol) formaldehyde and chromatin DNA was purified and digested by using SimpleChIP Enzymatic Chromatin IP Kits (Cell signaling) according to the manufacturer's instructions. Anti-p-CREB Ser133 antibody (Cell Signaling) and anti-CRTC2 anti-sera were used for immunoprecipitation. Precipitated DNA was quantified by real-time PCR (primer sets in Supplementary Tables S2 and S3 ) and was calculated relative to input DNA. RNAi and nucleofection Mouse Creb1 , Crtc2 and scrambled control siRNA were obtained from Stealth RNAi (Invitrogen). The sequence of Creb1 siRNA: 5′-UUGAACAACAACUUGGUUGCUGGGC-3′ (sense) or 5′-GCCCAGCAACCAAGUUGUUGUUCAA-3′ (antisense); Crtc2 siRNA: 5′-GCCAUGGCUCAGGACCUAAUAUCAU-3′ (sense) or 5′-AUGAUAUUAGGUCCUGAGCCAUGGC-3′ (antisense). Freshly isolated CD4 + T cells were transfected with 500 pmol siRNA using Amaxa P3 Primary Cell 4D-Nucleofector X Kit with the programme DN100 on a 4D-Nucleofector (Lonza) in 100 μl. Cells were directly transferred into full RPMI1640, then were cultured and stimulated in the presence of IL-7. Alternatively, CD4 + T cells were preactivated with anti-CD3 and anti-CD28 for 2 days, then ‘rest’ on ice for 1–2 h followed by transfecting with 5 μg plasmids in 100 μl using Amaxa P3 Primary Cell 4D-Nucleofector X Kit with the programme EO115 on a 4D-Nucleofector (Lonza). Cells were then cultured and stimulated. Luciferase assay To determine the CRTC2 transcriptional activity, preactivated CD4 + T cells were nucleofected with GAL4-fusion pM-mCRTC2 and pTAL-5x GAL4-Luciferase reporter and pRL-TK renilla luciferase reporte as internal control and treated with db-cAMP as indicated. To construct the mouse Il12rb2 reporter vector, a 5′-upstream fragment from −4.4 kb to +70 bp of the mouse Il12rb2 promoter/enhancer region were cloned by PCR and inserted into the pGL4.17 luciferase reporter vector (Promega). The sequence of primers: 5'-CTATGCTGCTGCCTGAAAGATGAGG-3' (forward) and 5′-AGGGCACCTACCACTATCCTCATCC-3′ (reverse). EL4 cells stably expressing the mouse Il12rb2 reporter and the internal control renilla luciferase (Promega), EL4- Il12rb2 -luc cells, were stimulated with anti-CD3 (5 μg ml −1 ) and db-cAMP or vehicle for 24 h, then harvested for luciferase assay. Alternatively, EL4- Il12rb2 -luc cells were transfected with siRNA or plasmids followed by stimulation with anti-CD3 and db-cAMP as described in the figure legend. Luciferase activities in cell lysates were detected by The Dual-Luciferase Reporter Assay System (Promega). CHS model We sensitized Lck-Cre − EP4 fl/fl and Lck-Cre + EP4 fl/fl mice with 25 μl of 1% (w/v) DNFB in acetone/olive oil (4/1, v/v) on shaved abdominal skin on day 0. dLN cells of one mouse were collected on day 5, and then transferred into one naive B6 mouse. The recipient mice were immediately challenged by application of 20 μl of 0.3 or 0.5% DNFB to their ear, and ear thickness was measured with a micrometre for each mouse before and 24 h after elicitation, and the difference is expressed as ear swelling. Alternatively, the dLN cells were harvested from DNFB-sensitized mice on day 5 to detect mRNA or protein expression of cytokine receptors or were subjected to isolation of CD4 + T cells by antoMACS, and in vitro restimulated with anti-CD3 and anti-CD28 for 24 h for measuring cytokine production. Colitis model Adoptive transfer colitis model has been described [43] . Briefly, naive CD4 + CD25 − CD45RB hi T cells were prepared from Lck-Cre + EP4 +/+ or Lck-Cre + EP4 flox/+ mice by cell sorting. Cells (5 × 10 5 cells per mouse) were transferred intravenously into mice deficient in recombination-activating gene 2 ( Rag2 ). CD4 + T cells from mesenteric lymph nodes of each recipient mouse were purified by auto-MACS on day 42 after T-cell transfer and stimulated with anti-CD3 for 72 h. IFN-γ and IL-2 production in supernatants and gene expression in CD4 + T cells were determined by enzyme-linked immunosorbent assay and real-time PCR, respectively. Data analysis All data were expressed as mean±s.e.m., and statistical significance was examined by the unpaired two-tail Student’s t -test except where indicated, using GraphPad (Prism) or Excel (Microsoft). How to cite this article: Yao, C. et al . Prostaglandin E 2 promotes Th1 differentiation via synergistic amplification of IL-12 signalling by cAMP and PI3-Kinase. Nat. Commun. 4:1685 doi: 10.1038/ncomm2684 (2013).